Loss of frugivore seed dispersal services under climate change The capacity of species to track shifting climates into the future will strongly influence outcomes for biodiversity under a rapidly changing climate. However, we know remarkably little about the dispersal abilities of most species and how these may be influenced by climate change. Here we show that climate change is projected to substantially reduce the seed dispersal services provided by frugivorous vertebrates in rainforests across the Australian Wet Tropics. Our model projections show reductions in both median and long-distance seed dispersal, which may markedly reduce the capacity of many rainforest plant species to track shifts in suitable habitat under climate change. However, our analyses suggest that active management to maintain the abundances of a small set of important frugivores under climate change could markedly reduce the projected loss of seed dispersal services and facilitate shifting distributions of rainforest plant species. It is well understood that all species possess relatively fixed tolerances to environmental conditions (their fundamental niche [1] ) and that these tolerances are important in influencing the spatial distribution of species [2] . Under climate change, these physiological constraints imply that many species will need to shift their geographic distributions and track suitable habitats in order to persist [3] . Given these basic concepts, substantial research has focussed on understanding how the distributions of species may shift under climate change, through model projections [4] and long-term observations [5] . Modelling of current and future distributions indicate that some species will only persist by moving substantial distances in the coming century [6] . However, few studies have incorporated dispersal processes into understanding possible shifts in biodiversity under climate change [7] , despite the demonstrated importance of movement potential [8] , [9] , [10] . The sparse consideration given to dispersal stems from both the additional modelling effort required and the shortfalls in our knowledge of dispersal attributes for most species. The movement of organisms over space and time involves processes that are often complex and difficult to measure [11] , which has limited our knowledge of dispersal to a relatively small number of well-studied species [7] . Compounding the shortfalls in our knowledge of dispersal is the possibility that dispersal capacity itself may be markedly altered by climate change [12] , [13] . To date, this has been best studied for wind-dispersed temperate and boreal plant species, where the population spread of a species can be mechanistically modelled, accounting for environmental effects on physiology, demographic processes and physical seed movement [14] . Although these studies have not made spatially explicit projections, they show that climate change has the potential to both increase [14] , [15] and decrease [16] , [17] the capacity of different wind-dispersed plant species to shift their distributions over time. In more complex systems, such as tropical rainforests, the majority of plant species produce fleshy fruits and their seeds are dispersed by a variety of frugivorous vertebrates [18] . There is a strong likelihood that climate-induced changes in the abundance and distribution of these frugivores will lead to large changes in the seed dispersal services they provide [12] , [18] , [19] . Understanding the implications of climate change for seed dispersal in tropical forests has, however, been limited by the diversity of both plants and frugivores in these systems, with complex and changing interactions likely over both space and time [20] . Here we quantified the potential impacts of climate change on the dispersal services provided by 45 frugivorous vertebrates (birds, bats and arboreal marsupials) for 1,345 fleshy fruited tropical rainforest plant species in the Australian Wet Tropics. This region supports unique and diverse flora and fauna [21] , for which one of the worlds best data sets on tropical forest frugivory and seed dispersal has been assembled [22] , [23] , [24] , [25] . We applied these data to generate fine-resolution spatially explicit dispersal kernels for different plant fruit groups (PFGs) under both current and future (2100) climates. We also assessed the potential benefits for seed dispersal of actively maintaining the current abundances of different frugivorous vertebrates. Our analyses show substantial changes in dispersal kernels for the Australian Wet Tropics under climate change, with major reductions in both median and long-distance dispersal for most PFGs in most areas. We also demonstrate that these negative outcomes for dispersal capacity could be substantially ameliorated through management that would actively maintain the abundances of a small set of important frugivores. Although the present analyses make some simplifying assumptions (for example, ignoring climate change impacts on frugivore behaviour and physiology) and do not consider subsequent outcomes for plant diversity, they form a strong basis for improving our understanding of dispersal and biodiversity dynamics under climate change. Change in dispersal kernels Owing to the differential contribution of frugivorous vertebrates, projected dispersal kernels were complex, often varying markedly over space, time and between PFGs ( Fig. 1c–h ). Here we summarize these complex dispersal kernels using the median dispersal distance (50th percentile) and long-distance dispersal (99th percentile), which both have relevance for the capacity of plant species to spread under climate change [26] . The median dispersal distances for all PFGs across the Australian Wet Tropics ( Supplementary Fig. 1 ) were projected to decrease markedly under climate change ( Fig. 1 ; Supplementary Fig. 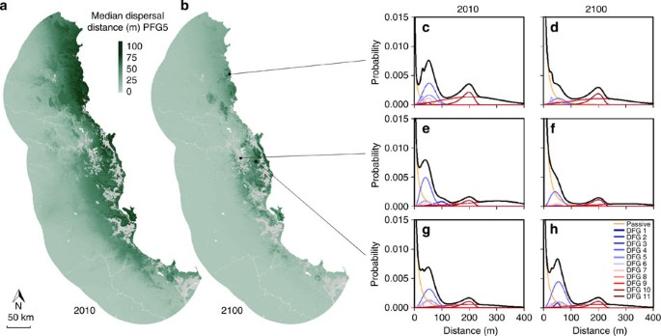Figure 1: Present and future seed dispersal in the Australian Wet Tropics. (a,b) Spatial projections of median dispersal distance for 2010 (a) and 2100 (b), for the most common plant fruit group (PFG5—small drupes), with human land-use in grey. Also shown are projected present and future dispersal kernels for PFG5 for three locations: Cedar Bay National Park (c,d), fragmented forest on the Atherton Tablelands (e,f) and the summit of Mt Bartle Frere (g,h). The contribution of different disperser functional groups (DFG) and passive dispersal to the total dispersal kernels (c–h) are also displayed. Note, the dispersal kernels extend beyond thexandy-values shown (c–h). 2 ; Supplementary Table 1 ). Although small and large fig fruits had the greatest current median dispersal distance (PFG1=100.6±49.6 m and PFG2=111.8±55.1 m; Supplementary Fig. 2a–d ; Supplementary Table 1 ) across the 224,733 grid cells, the largest relative loss in median dispersal distance under climate change was projected for plants with small multiple fruits (46.4% loss; Supplementary Fig. 2e,f ; Supplementary Table 1 ) and small drupes (46.9% loss; Fig. 1a,b ; Supplementary Table 1 ). Figure 1: Present and future seed dispersal in the Australian Wet Tropics. ( a , b ) Spatial projections of median dispersal distance for 2010 ( a ) and 2100 ( b ), for the most common plant fruit group (PFG5—small drupes), with human land-use in grey. Also shown are projected present and future dispersal kernels for PFG5 for three locations: Cedar Bay National Park ( c , d ), fragmented forest on the Atherton Tablelands ( e , f ) and the summit of Mt Bartle Frere ( g , h ). The contribution of different disperser functional groups (DFG) and passive dispersal to the total dispersal kernels ( c – h ) are also displayed. Note, the dispersal kernels extend beyond the x and y -values shown ( c – h ). Full size image We summarized the results across the seven PFGs by calculating the average median or long dispersal distance for each location, where the contribution of each PFG to the average was weighted by the proportion of the fleshy fruited flora within that PFG ( Table 1 ). This synthetic analysis revealed widespread and substantial reductions in median dispersal distance under climate change, with 97.2% of the Wet Tropics bioregion projected to have lower median dispersal distances in 2100 ( Fig. 2a ). The greatest reductions in median dispersal distance were projected for rainforest currently occurring in lowland areas and on the western margin ( Fig. 2a ). Loss of dispersal services in these areas under climate change is associated with marked reductions in the predicted environmental suitability for important vertebrate frugivores in the region, resulting in decreased abundances. Table 1 The DFG that could best promote median and long-distance dispersal for each PFG to 2100 under climate change. 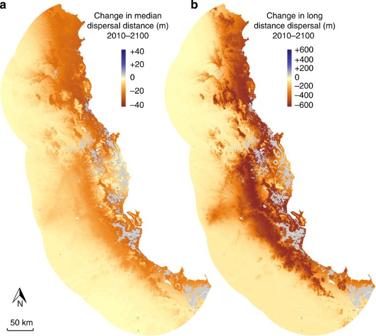Figure 2: Projected change in median and long-distance dispersal under climate change. (a,b) Spatial projection of change in the median (50th percentile) dispersal distance (a) and long-distance dispersal (99th percentile) (b) from 2010 to 2100 under climate change. Data are a weighted mean across all plant fruit groups in the Australian Wet Tropics, with human land-use shown in grey. Full size table Figure 2: Projected change in median and long-distance dispersal under climate change. ( a , b ) Spatial projection of change in the median (50th percentile) dispersal distance ( a ) and long-distance dispersal (99th percentile) ( b ) from 2010 to 2100 under climate change. Data are a weighted mean across all plant fruit groups in the Australian Wet Tropics, with human land-use shown in grey. Full size image We project substantial reductions in long-distance dispersal for fleshy fruit plant species, with decreases across 99.5% of the Wet Tropics bioregion ( Fig. 2b ). The spatial nature of the projected change in long-distance dispersal to 2100 was very similar to that for median dispersal distance ( Fig. 2a ); however, loss of long-distance dispersal was not distributed evenly between PFGs. For example, we project 52–56% decrease in the long-distance dispersal of small fruits (PFG1, PFG3 and PFG5), but minimal loss (≤5%) of long-distance dispersal for larger fruits (PFG2, PFG4 and PFG6) ( Supplementary Table 1 ). Although we project overall loss of dispersal services in the Australian Wet Tropics under the worst-case climate scenario, median and long dispersal distances of some PFGs in some areas were projected to increase into the future. The greatest projected local gains in median dispersal distance under climate change were for fig fruits (PFG1 and PFG2), which increased by >100 m in higher elevation rainforests ( Supplementary Fig. 2a–d ; Supplementary Table 1 ). Indeed, we found significant increases in median and long-distance dispersal above 1,300 m elevation for all PFGs ( Fig. 2 ; Supplementary Fig. 3 ). Sensitivity analyses To understand the sensitivity of our dispersal kernel projections to the underlying parameters ( Supplementary Tables 2 and 3 ), we performed a one-at-a-time sensitivity analysis for the five major parameter sets (abundance, proportion fruit eaten, passive dispersal, gut passage time and displacement). This analysis indicated that current median dispersal distances were more sensitive to variation in the gut passage time and displacement parameter sets, than to the parameters for estimating frugivore abundance from predicted habitat suitability, or those describing the proportion of fruit crop eaten per unit abundance ( Supplementary Fig. 4a ). These results were also broadly reflected in the projections for each PFG, although variation in parameter sets had contrasting effects on the magnitude of median dispersal distance for different PFGs ( Supplementary Table 4 ). In contrast, variation in the five parameter sets had roughly equivalent influence on long-distance dispersal ( Supplementary Fig. 4b ). Management for dispersal services Management actions that maintain the current abundances of the disperser functional group (DFG) 7 (throughout landscape frugivores) were projected to best promote median dispersal distances under climate change to 2100, by 7.4±2.7 m over all PFGs across the 224,733 grid cells ( Table 1 ). In contrast, managing the abundances of DFG11 (wide-ranging, slow gut frugivores) was found to best promote long-distance dispersal under climate change, by 451.7±140.5 m across all PFGs across the 224,733 grid cells ( Table 1 ). There was little consistency across PFGs in terms of which DFG would best promote median or long dispersal distances under climate change ( Table 1 ). In addition, maintaining the abundances of some DFGs under climate change could actually reduce median or long dispersal distances for some PFGs ( Supplementary Table 5 ). The projected effects of actively maintaining frugivore abundances under climate change also varied spatially over the Australian Wet Tropics. For example, maintaining the abundances of frugivore species within DFG11 (wide-ranging, slow gut frugivores) increased the long-distance dispersal of PFG3 (small multiple fruits) under climate change by 990.1 m on average across the 224,733 grid cells ( Table 1 ), but by up to 1,447 m along the western margin of the current rainforest ( Fig. 3 ). 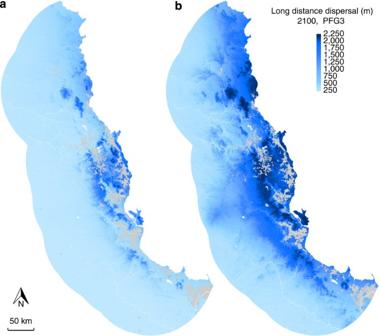Figure 3: Potential benefits for long-distance dispersal in maintaining abundances of ‘wide-ranging slow gut’ dispersers (DFG11) under climate change. (a,b) Spatial projection of long-distance dispersal (99th percentile) in 2100 under climate change for plant fruit group 3 (PFG3—small multiple fruits). Projections assume either no ameliorative management of vertebrate disperser abundances (a), or that abundances of disperser functional group 11 (wide-ranging slow gut) are maintained at 2010 levels through active management (b). Human land-use is shown in grey. Figure 3: Potential benefits for long-distance dispersal in maintaining abundances of ‘wide-ranging slow gut’ dispersers (DFG11) under climate change. ( a , b ) Spatial projection of long-distance dispersal (99th percentile) in 2100 under climate change for plant fruit group 3 (PFG3—small multiple fruits). Projections assume either no ameliorative management of vertebrate disperser abundances ( a ), or that abundances of disperser functional group 11 (wide-ranging slow gut) are maintained at 2010 levels through active management ( b ). Human land-use is shown in grey. Full size image Climate change is likely to cause major alterations to the distributions and abundances of species as well as the composition of communities [10] , [27] , [28] . Here we have demonstrated that for the Australian Wet Tropics, climate-induced changes in frugivore abundances may well flow through and substantially alter the seed dispersal services they provide, hence influencing outcomes for the rainforest flora under climate change. Our analyses showed loss of seed dispersal services over most of the Australian Wet Tropics, with median dispersal distances decreasing by 38.7% to 2100 ( Fig. 2 ). Importantly, not all PFGs were projected to be impacted equally ( Supplementary Fig. 2 ). The two most common PFGs in the Australian Wet Tropics (small multiple fruits and small drupes) were projected to suffer the greatest reduction in median dispersal distances ( Supplementary Table 1 ), implying that large numbers of tropical forest plant species will find it increasingly difficult to track rapid shifts in suitable climates. Although median dispersal distance is a useful measure for characterizing dispersal kernels, it is now well recognized that rare long-distance dispersal events play a crucial role in influencing the geographic distribution of species and the capacity of populations to spread under changing climates [14] , [15] , [29] . Frugivorous vertebrates can be particularly effective in facilitating the long-distance dispersal of seeds, given the large movements some frugivores are capable of within the time taken for the seeds to travel through their gut [24] , [25] . Again, we project that plant species with small fruits will suffer the greatest reductions in long-distance seed dispersal under climate change (52–56%) with minimal loss (≤5%) of long-distance dispersal for larger fruits ( Supplementary Table 1 ). These contrasting changes in long-distance dispersal over time may well contribute to large compositional changes in tropical forest plant communities under a rapidly changing climate, with benefits for the spatial distributions of some species over others [27] , [30] . Our analyses provide a novel demonstration of why a spatially explicit consideration of dispersal under climate change is particularly important. For example, although we project climate-induced reductions in seed dispersal distances across most of the Australian Wet Tropics, we found significant increases in median and long-distance dispersal above 1,300 m elevation for all PFG’s ( Fig. 2 ; Supplementary Fig. 3 ). Increases in seed dispersal services at higher elevations under climate change are consistent with upslope shifts in the distribution and abundances of vertebrate frugivore species under climate change, as predicted here and found in other studies [5] , [31] . These increases in dispersal at higher elevations over time may facilitate concomitant upslope shifts in the distributions of the rainforest flora under a warming and drying climate [32] . Given the large threat that climate change poses to seed dispersal in the Australian Wet Tropics ( Figs 1 and 2 ), it may be appropriate to consider management options that promote seed dispersal services, facilitating rainforest plant species to shift their distributions over time. Here we assessed a simple hypothetical management strategy of actively maintaining the abundances of vertebrate frugivore species at their current levels into the future as the climate changes. Strategies aiming to promote the abundances of animal species have been implemented over a long history of conservation management and include both simple approaches (for example, providing food/water supplement and controlling alien predators) [33] , [34] as well as those requiring higher levels of investment (for example, captive breeding and translocation) [35] , [36] . Our analyses demonstrate that there are a wide range of possible benefits for dispersal services by sustaining the abundances of different frugivores and these benefits can vary markedly between PFGs ( Table 1 ; Supplementary Table 5 ). Not only did different DFGs best retain dispersal services for different PFGs ( Table 1 ), but management actions that maintained the abundances of some DFGs under climate change could actually result in decreased dispersal distances compared with no management ( Supplementary Table 5 ). This finding adds weight to arguments that active species management under climate change needs to adequately consider the consequences for both other species and broader ecosystem processes [37] . Projections from studies such as ours could help identify the consequences of conservation actions on important ecosystem processes, as well as highlight in which areas seed dispersal services could benefit most by active management of frugivore populations into the future ( Fig. 3 ). Our analyses highlight the complexity of frugivore-mediated seed dispersal, especially when considered in a spatially explicit manner for a diverse system undergoing large environmental changes [12] , [18] , [19] . This inherent complexity leads to multiple aspects of our analyses possessing substantial uncertainty, including our projections of current and future species abundances ( Supplementary Table 2 ), current and future frugivore movement behaviour and fruit consumption patterns ( Supplementary Table 3 ), potential invasions by alien frugivore species, plus broader issues, such as uncertainty in climate projection, human land-use change, plant community dynamics and the adaptive potential of frugivores to environmental change. Further, there are important processes that we have not incorporated into our analyses, such as demographic processes of frugivore populations, or potential climate-induced changes in behaviour and physiology. Given these uncertainties, our study applies best available understanding of current and future seed dispersal services in the Australian Wet Tropics, synthesized from one of the best available community-level data sets on frugivore-mediated seed dispersal [22] , [23] , [24] , [25] . Our projected dispersal kernels were most sensitive to variation in the parameters associated with passive dispersal, gut passage time and frugivore displacement ( Supplementary Fig. 4 ; Supplementary Table 4 ), so further empirical research to refine these parameter sets is likely to contribute strongly to reducing the uncertainty of our dispersal projections. Undoubtedly this modelling and validation can be improved, as further data are collected, however, the relatively modest sensitivity of the dispersal projections to parameter variations suggests that the predictions of reduced seed dispersal services under climate change are robust. In less well-studied regions, it is possible that similar projections could be achieved by combining available information with data from similar taxa in other areas and mechanistic models of frugivore movement [38] . Here we have projected potential dispersal kernels across the Australian Wet Tropics for plant species of all fruit types, regardless of where those species actually occur now or in the future ( Figs 1 and 2 ; Supplementary Fig. 2 ). The spatiotemporal nature of the actual seed dispersal for each plant species will obviously depend on, and interact with, the spatial distribution of populations within each species, their demographics and their response to climate change. Future research could build on our results by quantitatively assessing the possible implications of the projected changes in dispersal kernels on outcomes for tropical forest plant species and communities under climate change. This may include application of recently developed dynamic macroecological modelling techniques [27] to assess climate change outcomes across the entire flora of the Australian Wet Tropics. Although our results are directly relevant to the Australian Wet Tropics, they also have broader implications for rainforests globally, as well as other systems where frugivores influence seed dispersal. In such systems, rapid climate change is likely to substantially alter the composition of frugivore communities, changing seed dispersal services and subsequent plant movement capacity. Our analyses have demonstrated that these changes can at least partially be ameliorated through strategic management of frugivore abundances under a changing climate. Analytical approach For each important frugivore species in the Australian Wet Tropics ( n =45), we predicted their current and future abundance by modelling their habitat suitability using MaxEnt [39] and converting predicted habitat suitability of each species to abundance using existing correlative relationships [40] ( Supplementary Table 2 ). This included a number of frugivore species that are currently less common in the Australian Wet Tropics, but may become more abundant across the region under climate change. We examined a single climate future (A1FI emissions scenario in CSIRO mk3.5 GCM) that represents a ‘worst-case scenario’ for biodiversity in the Australian Wet Tropics (greatest projected warming and drying to 2100). In order to simplify the complexity of possible plant–frugivore interactions and allow data gaps to be readily filled, we applied previously established trait-based functional groupings [22] , [23] for both plants (seven PFGs) and frugivores (11 DFGs). We then constructed spatially and temporally explicit dispersal kernels for each PFG, by combining projected current and future abundances of each disperser species with empirical data on their feeding preferences, movement behaviour and gut passage time [22] , [23] , [24] , [25] ( Supplementary Fig. 5 ; Supplementary Table 3 ). To account for the potential effects of habitat fragmentation influencing seed dispersal by frugivorous vertebrates [19] , [41] , we also applied data on movement behaviour in fragmented habitat in generating dispersal kernels, with fragmented areas spatially defined and assumed to remain constant over time ( Supplementary Fig. 6 ). Projecting current and future frugivore abundances To generate habitat suitability models for the 45 vertebrate frugivore species that were robust to projection under climate change, models were developed using occurrence and environment data from across all Queensland ( Supplementary Fig. 1b ), before being projected to the smaller Australian Wet Tropics study region at 250 m resolution ( Supplementary Fig. 1c ). The environment data applied in the models included 12 environmental variables hypothesized or previously found to be important in influencing the spatial distribution of vertebrates in the Australian Wet Tropics [31] , [40] , with all 12 variables being included in the models for each frugivore species ( Supplementary Table 2 ). Current and future environmental layers were derived at 250-m grid resolution using ANUCLIM v6.1 (ref. 42 ), with radiation corrected for slope and aspect. Occurrence data for the 45 vertebrate frugivores were obtained from the Atlas of Living Australia and the Queensland Government’s WildNet database, with records only used in generating the habitat suitability models if they were both recent (after 1990) and spatially accurate (<300 m uncertainty) ( Supplementary Table 2 ). To further promote the development of models that were robust to projecting habitat suitability under climate change, we applied only linear, quadratic and product responses in fitting models with MaxEnt [39] , to avoid over-fitting models to current distribution patterns [43] . We applied default settings for MaxEnt model regularization, as suggested by Phillips and Dudik [44] , and implemented a 10-fold cross-validation to assess predictive performance. In projecting future habitat suitability under climate change, we assumed no limitations in the capacity of frugivores to move to suitable habitat, which is likely to be the case for most of the frugivores considered here. To convert the predicted habitat suitability of each species to abundance, we applied correlative negative exponential models previously derived [40] , using either mean parameter values of the nearest taxonomic group or literature values for those species for whom no models relating habitat suitability to abundance were available ( Supplementary Table 2 ). While we have attempted to produce robust predictions of shifts in the abundances of frugivore species under climate change, as with other applications of species distribution modelling, these ignore potentially important processes, such as interspecific interactions and genetic adaptation. Constructing spatiotemporally explicit dispersal kernels To construct spatially and temporally explicit dispersal kernels for each PFG, we combined the projected abundances of each disperser species with data and functions summarizing the feeding preferences, movement behaviour and gut passage time of each DFG ( Supplementary Fig. 5 ). Available movement data for species in each DFG in both contiguous and fragmented habitat [22] , [25] were used to model displacement ( d , in metres) over time ( t , in minutes), using a two-parameter negative exponential function: where c and z are fitted parameters, which differ between fragmented and contiguous habitat ( Supplementary Table 3 ). Of a variety of models assessed, the negative exponential function was selected owing to its simplicity and accuracy in representing the displacement data available. Available data [22] , [25] on the gut passage time for a wide range of PFGs eaten by frugivore species within each DFG were used to model the probability of a seed exiting the gut over time ( P ( t )), using the gamma distribution [38] : where with k and θ being the fitted parameters. The gamma distribution is commonly applied in describing the time taken for seeds to pass through animal digestive systems [38] , [45] . Models of displacement and gut passage time were significant for all DFG’s ( P <0.001). Data on the proportion of the fruit crop of each PFG eaten by each DFG across 42 locations in the Australian Wet Tropics were related to observed abundances within each DFG to obtain estimates of the proportion of the plant fruit crop eaten per unit DFG abundance ( Supplementary Table 3 ). These data were obtained through focal tree observations documenting 6,109 frugivory interactions between 73 fruiting plant species and 46 frugivore species [22] , [23] , [25] . Here we assume that our estimates of the proportion of fruit crop eaten per unit frugivore abundance ( Supplementary Table 3 ) remains constant into the future, which is the simplest assumption possible given the lack of long-term data on frugivory interactions. Where movement, gut passage or frugivory data for a DFG were not available, parameters for the functionally closest DFG were applied. For fruit remaining uneaten, we modelled passive dispersal using the two-dimensional negative square power law model [46] , [47] : where Pd i,j is the probability of dispersal from location i to j , r ij is the radial distance between i and j , λ is the median dispersal distance (here we use 5 m [26] ), and K is the scaling factor (here K =13). The negative square power law model has a ‘fat tail’ distribution, making it suitable for representing rare long-distance passive dispersal events [46] , [48] . For each PFG in each grid cell, a complete (stacked) dispersal kernel (for example, Fig. 1c–h ) was calculated by apportioning fractions of the fruit crop to each DFG based on their predicted proportion of fruit crop eaten in that grid cell, with the fraction of fruit uneaten allocated as passive dispersal ( Supplementary Fig. 5 ). Sensitivity analyses While the spatially and temporally explicit dispersal kernels we have constructed are based on the best available knowledge and data on frugivore-mediated seed dispersal in the Australian Wet Tropics, substantial uncertainty remains in terms of the parameter values we have estimated and applied. Indeed, for many of the parameters, there is insufficient information to properly characterize the range or probability distribution of possible values. Hence, here we apply a simple one-at-a-time sensitivity analysis to assess which set of parameters most strongly influence the projected dispersal kernels [49] . First we grouped the parameters into five sets: those associated with estimating the abundance of each frugivore species given their predicted habitat suitability (abundance coefficient and maximum abundance in Supplementary Table 2 ); those describing the proportion of fruit crop eaten per unit frugivore abundance ( Supplementary Table 3 ); those describing passive dispersal of uneaten fruit ( λ and K above); those describing the gut passage time for each DFG ( k and θ in Supplementary Table 3 ); and those describing the displacement of each DFG ( c and z in Supplementary Table 3 ). For each set of parameters in turn, we varied all parameters in that set 100 times by selecting an alternative value, in a uniform random manner, from the range±50% of its estimated value. We applied the same range (±50%) for each parameter, given limited information regarding the likely distribution of parameters and to standardize the effect of parameter variation between parameter sets. We then calculated current dispersal kernels for each PFG across the Wet Tropics bioregion as described above, determined the median dispersal distance (50th percentile) and long-distance dispersal (99th percentile) for each PFG in each grid cell, with the averages of these for each PFG across all grid cells used as the output value for the sensitivity analysis. Assessing management of frugivores under climate change We assessed the potential benefits for seed dispersal in actively maintaining the current abundances of different frugivorous vertebrates. We constructed current (2010) and future (2100) dispersal kernels, as in our original analyses, but separately maintained the current abundances of the species within each DFG constant into the future, as a simple approximation of management activities that maintain frugivore populations under climate change [37] . How to cite this article: Mokany, K. et al. Loss of frugivore seed dispersal services under climate change. Nat. Commun. 5:3971 doi: 10.1038/ncomms4971 (2014).